Interspecific bacterial sensing through airborne signals modulates locomotion and drug resistance Bacteria use chemical signals to sense each other and to regulate various physiological functions. Although it is known that some airborne volatile organic compounds function as bacterial signalling molecules, their identities and effects on global gene expression and bacterial physiological processes remain largely unknown. Here we perform microarray analyses of Escherichia coli exposed to volatile organic compounds emitted from Bacillus subtilis . We find that 2,3-butanedione and glyoxylic acid mediate global changes in gene expression related to motility and antibiotic resistance. Volatile organic compound-dependent phenotypes are conserved among bacteria and are regulated by the previously uncharacterized ypdB gene product through the downstream transcription factors soxS , rpoS or yjhU . These results strongly suggest that bacteria use airborne volatile organic compounds to sense other bacteria and to change master regulatory gene activity to adapt. Many bacterial species co-exist in dynamic communities where they compete or cooperate with one another [1] , [2] , in the regulation of their functions [3] , [4] , [5] . Bacteria have developed intercellular signalling systems to adapt to natural variations caused by stress, competition and countering host defenses [6] . Several bacterial communication pathways have been discovered [7] . The most widespread phenomenon is quorum sensing (QS), which is an interconnected, multi-layered regulatory network that includes the secretion of QS molecules [8] , [9] and their concentration-dependent signalling cascades [10] . Bacteria perform QS with chemicals, such as N -acyl derivatives of homoserine lactone, cyclic dipeptides and quinolones [10] , [11] , [12] , [13] , [14] , to sense and respond to external and internal signals, and environmental cues. More than 300 bacteria release a wide variety of biologically active airborne volatile organic compounds (VOCs) that can diffuse in heterogeneous mixes of solids, liquids and gasses [15] , [16] , suggesting that VOC production is a general phenomenon of bacteria. However, the mechanisms underlying VOC-mediated bacterial communication, the identities of active VOCs and the cellular behaviours that are affected remain largely unknown, except in some cases. For example, in the opportunistic human pathogen Pseudomonas aeruginosa , the 2-aminoacetophenone VOC modulates virulence regulator activity and promotes a bistable phenotype by stochastically silencing acute virulence functions [12] . More directly, VOCs modify the antibiotic resistance phenotype of Escherichia coli [13] , [14] . It is becoming clear that VOCs have a role in interkingdom interactions between bacteria and eukaryotic cells. For example, Vibrio cholerae O1 produces the gaseous compound 2,3-butanediol, which interacts with the human immune system by suppressing the induction of immune modulators [17] . Bacterial VOCs also have been shown to promote plant growth [18] and induce systemic resistance in Arabidopsis [19] . Therefore, the roles played by bacterial VOCs and their functional mechanisms need to be elucidated fully to develop a wider understanding of bacterial survival in dynamic multitrophic interactions. The structures of Gram-negative and Gram-positive bacteria appear significantly different, but recent metagenomics studies showed that both bacterial species co-exist in any natural habitats, such as human, soil or wate, with different populations [20] , [21] , [22] , [23] . The abilities of these bacteria to communicate and respond to different environmental conditions could be major factors in making a large and dynamic bacterial community. There are many potential trade-offs for communications between two bacterial groups that allow bacteria to co-exist and maintain their own survival in variable environments. However, it is technically challenging to experimentally study bacterial communications in variable environments. The two species E. coli and Bacillus subtilis are known to share similar ecological niches [20] , [21] , [22] . In this study, E. coli and B. subtilis were used as representative models for studying the roles and effects of VOCs in Gram-negative and Gram-positive species, respectively. Microarray analysis was used to examine gene expression in E. coli in response to exposure to VOCs from B. subtilis , to understand how these VOCs affect the intercellular regulation of gene expression. VOCs dramatically affected the phenotypes of receiver cells and altered the expression of more than 100 genes. Treatment with 2,3-butanedione (2,3-BD) and glyoxylic acid (GA) in nanomolar to micromolar concentrations mediated changes in global gene expression that correlated with motility and antibiotic resistance phenotypes. VOC-mediated interactions were modulated by the previously uncharacterized ypdB gene product and its downstream transcription factors, soxS , rpoS or yjhU . The results of this study strongly suggest that VOCs represent a cross-specific signal for rapid sensing between bacteria that triggers variations in gene expression. VOC-mediated bacterial communication may induce modifications that affect the self-defence and motility of physically separated bacteria. B. subtilis VOCs alter the expression of E. coli genes A model system was designed to examine the mechanisms underlying phenotypic modifications induced by bacterial metabolites in interspecies interactions. B. subtilis 168 (ref. 24 ), and E. coli K12 strains were used as emitter and receiver bacteria, respectively. B. subtilis produces diffusible secondary metabolites, such as antibiotics and VOCs [25] . These products can affect plant defence systems by eliciting innate immunity against a broad spectrum of pathogens [18] , [19] . It was hypothesized that the VOCs produced by B. subtilis modulate the expression profiles and functions of certain E. coli genes. A two-compartment Petri plate (I-plate) assay was used for concurrent growth of bacteria ( Fig. 1a ). In this assay, E. coli grown on Luria-Bertani (LB) agar was exposed to VOCs from B. subtilis 168 cell suspensions grown on tryptic soy broth (TSB) agar. There was no physical contact between the cultures or the bacteria. E. coli cells were collected after different periods of exposure to VOCs (6, 12 and 24 h), and transcription profiling of E. coli gene expression was performed using microarray analyses of 4,440 open-reading frames. The 6-, 12- and 24-h treatments showed differential expression of 137, 569 and 93 genes (>3-fold change), respectively ( Supplementary Table S1 ). The largest change in gene expression occurred after 12 h of exposure to B. subtilis VOCs. To confirm the responses of these genes to B. subtilis VOCs, three of the top 50 genes identified by microarray analysis ( ycfR , aaeX and hyaF ) were selected for further analysis. Gene expression was examined by reverse transcription quantitative PCR (RT–qPCR). As expected, all three genes showed increased expression in response to B. subtilis VOCs ( Fig. 1b ), with ycfR exhibiting the greatest change. Further analyses were performed using the Gene Ontology website tools [26] ( Supplementary Table S1 ) or Kyoto Encyclopedia of Genes and Genomes [27] information. Strongly affected genes were allocated into functional groups, such as motility, peptide transport, toxin-antitoxin (TA) system, protein synthesis, polyamine metabolism and sugar transport ( Fig. 1c , Supplementary Table S2 ). To validate the microarray data, two different transcripts were selected from each group, and expression profiles were determined by RT–qPCR. These data closely matched the Gene Ontology patterns of the microarrays ( Fig. 1d ). Thus, the microarray results identified E. coli genes modulated by B. subtilis VOCs. Their functional clusters may shed light on the mechanisms underlying the physiological responses of this receiver. 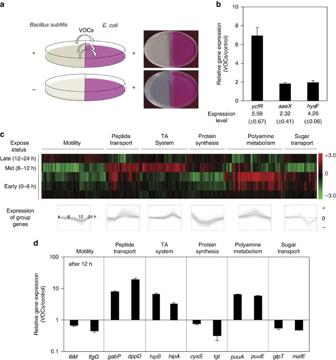Figure 1: Effect ofB. subtilisVOCs onE. coligene expression. (a) Schematic showing the two-compartment plate assay (I-plate system). For growth ofE. coli, LB agar was used; for visualization and photography, MacConkey-agar plate was used. (b) Relative gene-expression analysis ofE. coli. Three genes showing >3-fold changes in expression in response toB. subtilisVOCs in microarray data are represented as ‘Expression level’; these were randomly selected and analysed by RT–qPCR afterE. colicells were treated with VOCs for 12 h. Error bars are defined as s.e.m. (n=3,P=0.05). (c) Clustering of microarray data. The microarray data show >3-fold up- or downregulation induced by treatment with VOCs. Clustering analysis was performed using MultiExperiment Viewer45. Three treatment periods are shown (6, 12 and 24 h) (d) Gene-expression pattern of clustered groups. Two genes were randomly selected from each of the groups incand examined by RT–qPCR using gene-specific primers listed inSupplementary Table S6. Error bars are defined as s.e.m. (n=3,P=0.05). Figure 1: Effect of B. subtilis VOCs on E. coli gene expression. ( a ) Schematic showing the two-compartment plate assay (I-plate system). For growth of E. coli , LB agar was used; for visualization and photography, MacConkey-agar plate was used. ( b ) Relative gene-expression analysis of E. coli . Three genes showing >3-fold changes in expression in response to B. subtilis VOCs in microarray data are represented as ‘Expression level’; these were randomly selected and analysed by RT–qPCR after E. coli cells were treated with VOCs for 12 h. Error bars are defined as s.e.m. ( n =3, P =0.05). ( c ) Clustering of microarray data. The microarray data show >3-fold up- or downregulation induced by treatment with VOCs. Clustering analysis was performed using MultiExperiment Viewer [45] . Three treatment periods are shown (6, 12 and 24 h) ( d ) Gene-expression pattern of clustered groups. Two genes were randomly selected from each of the groups in c and examined by RT–qPCR using gene-specific primers listed in Supplementary Table S6 . Error bars are defined as s.e.m. ( n =3, P =0.05). Full size image VOCs change the expression of motility-related genes From microarray data, VOC treatments decreased the expression of all 30 genes related to chemotaxis or the motility phenotype of E. coli ( Fig. 1d , Supplementary Tables S1 and S2 ). Motility-related genes are one of the key clusters associated with VOC-mediated physiological changes. Examination of the expression of some motility genes ( motA , cheA , cheW and fliA ) using RT–qPCR confirmed the microarray data ( Fig. 2a ). To verify the gene-expression changes correlated with the motility phenotype, the swimming and swarming abilities of VOC-treated E. coli cells were measured. Both swimming ( Fig. 2b ) and swarming ( Fig. 2c ) decreased by ~32% and ~60%, respectively. To test whether this phenotype is limited to E. coli or if it is a general trait of bacteria, B. subtilis VOCs were used to treat other Gram-negative bacteria, such as Burkholderia glumae BGR1 and P. aeruginosa PA14, and the Gram-positive bacteria Paenibacillus polymyxa E681. The swarming motility of each receiver bacteria was measured as a representative of motility phenotype. 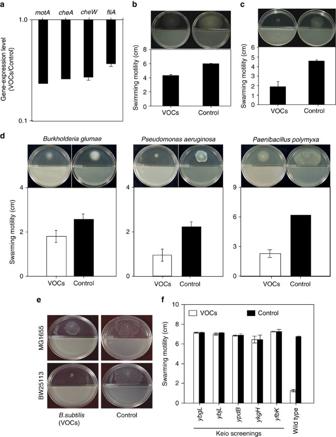Figure 2: Effect of VOCs on bacterial motility. (a) Change of motility-related gene expression. The expression of genesmotA,cheA,cheWandfliAinE. coliMG1655 was measured by RT-qPCR after treatment with VOCs. The gene-expression level indicates the normalized gene level of VOC-treated sample to non-treated sample (control). The data shown are the averaged values (n=5,P=0.05). Error bars are defined as s.e.m. VOC-induced changes in (b) swimming and (c) swarming motility ofE. coli. (d) Conservation of swarming motility in Gram-negative and Gram-positive bacteria. (e) Comparison of swarming motility in two differentE. colistrains. The plates are representative of data obtained in triplicate. (f)E. colimutant strains in which swarming motility was unchanged by VOCs.Supplementary Table S1contains further information about these genes. Figure 2d shows that swarming motility for all the species tested was decreased by VOCs, suggesting that VOCs are the general signalling molecules for altering bacterial motility. Because swarming ability was more strongly affected by VOCs than swimming ability, the changes to swarming activity were examined in greater detail. Figure 2: Effect of VOCs on bacterial motility. ( a ) Change of motility-related gene expression. The expression of genes motA , cheA , cheW and fliA in E. coli MG1655 was measured by RT-qPCR after treatment with VOCs. The gene-expression level indicates the normalized gene level of VOC-treated sample to non-treated sample (control). The data shown are the averaged values ( n =5, P =0.05). Error bars are defined as s.e.m. VOC-induced changes in ( b ) swimming and ( c ) swarming motility of E. coli . ( d ) Conservation of swarming motility in Gram-negative and Gram-positive bacteria. ( e ) Comparison of swarming motility in two different E. coli strains. The plates are representative of data obtained in triplicate. ( f ) E. coli mutant strains in which swarming motility was unchanged by VOCs. Supplementary Table S1 contains further information about these genes. Full size image To understand how the phenotype is modulated, the genes affecting the phenotype need to be identified. Therefore, a mutant library of E. coli genes [28] was screened to evaluate the effect of VOCs on the swarming motility. Because the Keio collection was developed from the strain E. coli BW25113 [29] , and different E. coli strains showed different motilities [30] , the effect of VOCs on the swarming motility of phenotypes using MG1655 [31] needed to be compared with that of BW25113 to show a general phenotype of E. coli. Exposure to VOCs caused a significant reduction in the swarming motility of E. coli BW25113 and MG1655 ( Fig. 2e ), suggesting that the effect is a general phenotype of E. coli . Therefore, BW25113 cells were used to validate the motility-related genes examined in Fig. 2e . Mutants of motA , che A, cheW and fliA showed no motility variation when the cells were exposed to VOCs, which suggests that they are essential for swarming ability ( Supplementary Fig. S1 ). However, the lack of motility in these mutants was similar to that of VOC-treated wild type. To identify a possible regulatory gene responsible for the VOC-mediated changes in swarming ability, mutants from the Keio collection were screened to identify knockouts of VOC-mediated genes that showed no significant variation in swarming motility with or without VOC treatment. Five mutants ( ybgL , ybjL , ypdB , ykgH and yfbK ) were identified ( Fig. 2f , Table 1 ). These data suggest that VOCs affect E. coli motility via previously uncharacterized motility-related genes. Table 1 Genes affecting VOC-dependent swarming motility. Full size table Antibiotic-resistance phenotype is mediated by TA genes From the microarray data, 27 different TA-related modules ( Supplementary Table S2 ) were upregulated by VOCs. The toxins relE (5.9-fold), yafQ (7.8-fold) and yoeB (6.8-fold) were strongly induced in persister cells [32] , [33] , [34] . Stationary-phase cultures of E. coli with hipBA , a representative TA system, represented a subpopulation of bacteria (~1% in the stationary state) that were viable after treatment with lethal concentrations of antibiotics [35] . Many bacterial VOCs modulate antimicrobial activity [36] , [37] , [38] . Therefore, we hypothesized that Bacillus VOCs could modulate multidrug resistance. First, the effect of VOCs on persister cells was analysed with respect to susceptibility to 240 commercial antibiotics. For this purpose, we used the Phenotype Microarray (PM) technique, which is a high-throughput technology for simultaneous testing of a large number of cellular phenotypes. It uses preconfigured well arrays of different cellular phenotypes and an automated instrument that monitors and records the response of cells in all wells of the arrays [39] . The effect of B. subtilis VOCs on the susceptibility of E. coli to different antibiotics varied ( Supplementary Fig. S2 ). Although VOCs exerted a marked effect on bacterial cells exposed to the PM12 plate, they did not improve resistance to all the antibiotics tested ( Fig. 3a ). 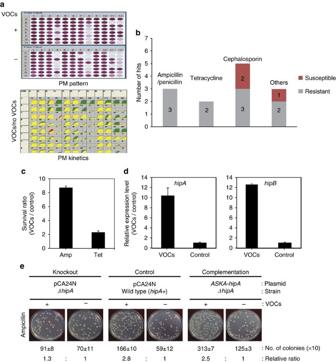Figure 3: Modulation of susceptibility to antibiotics by VOCs. (a) Representative kinetic analysis of antibiotic susceptibility ofE. colicells fromn=3 withP=0.05. PM pattern (left) and PM kinetics (right) of a PM12 plate. (b) Quantitative analysis of PM kinetics from PM11 to PM20. (c) Effect of VOCs on antibiotic resistance inE. coli. The relative survival ratio of VOC-treated to non-treatedE. coliin ampicillin or tetracycline is shown. (d) Expression ofhipAandhipBin the presence and absence of VOCs. Gene expression was monitored by RT-qPCR. Error bars are defined as s.e.m. from triplicate experiments. (e) Growth on ampicillin is dependent onhipAexpression. VOCs did not improve survival in thehipA-knockout strain, whereas VOCs improved survival in the complemented strain. The plasmids pCA24N and ASKA-hipAwere used50. Figure 3: Modulation of susceptibility to antibiotics by VOCs. ( a ) Representative kinetic analysis of antibiotic susceptibility of E. coli cells from n =3 with P =0.05. PM pattern (left) and PM kinetics (right) of a PM12 plate. ( b ) Quantitative analysis of PM kinetics from PM11 to PM20. ( c ) Effect of VOCs on antibiotic resistance in E. coli . The relative survival ratio of VOC-treated to non-treated E. coli in ampicillin or tetracycline is shown. ( d ) Expression of hipA and hipB in the presence and absence of VOCs. Gene expression was monitored by RT-qPCR. Error bars are defined as s.e.m. from triplicate experiments. ( e ) Growth on ampicillin is dependent on hipA expression. VOCs did not improve survival in the hipA -knockout strain, whereas VOCs improved survival in the complemented strain. The plasmids pCA24N and ASKA- hipA were used [50] . Full size image Thirteen antibiotics with Respiration Area >100 or <−100 were identified ( Supplementary Table S3 ) PM11 to PM20 plates. E. coli cells showed resistance to ten antibiotics and susceptibility to three antibiotics. Only the resistant phenotype was detected in the penicillin/ampicillin and tetracycline groups ( Fig. 3b ). These data suggest that resistance to antibiotics in these groups may be dependent on VOC treatment. The PM data were validated by growing VOC-treated and VOC-untreated E. coli on ampicillin and tetracycline. VOCs increased the number of ampicillin- and tetracycline-resistant cells by 8.7- and 2.3-fold, respectively ( Fig. 3c ). Microarray data ( Fig. 1 , Supplementary Table S1 ) showed that VOCs induced expression of hipA and hipB genes by 14.5- and 21.2-fold, respectively. VOC-mediated induction of these genes was confirmed by RT–qPCR ( Fig. 3d ). The expression of hipA is known to mediate persistence [40] . Mutant hipA7 cells show a very high frequency of persister formation, and overexpression of wild-type hipA confers persistence [41] , [42] , [43] . The effect of VOCs on ampicillin resistance in E. coli was examined with respect to expression of hipA to determine if hipA has a role in the VOC-mediated resistance phenotype. VOCs increased the number of wild-type cell colonies growing on ampicillin by 2.8-fold, but this effect was not observed in the hipA -deletion strain with control plasmid, in which the number of ampicillin-resistant colonies was reduced by ~30% ( Fig. 3e ). This effect was fully complemented in the knockout strain by an overproducer of hipA , which suggests that hipA is the necessary factor for regulating VOC-induced antibiotic resistance. These results indicate that, although TA-related genes are involved in VOC-dependent antibiotic resistance, additional cellular factors must be identified to develop a full understanding of the VOC-induced TA system. Identification of VOCs that affect bacterial phenotypes B. subtilis emits ~30 different VOCs [44] , but how many or which specific VOCs modulate newly identified phenotypes remains to be validated. Therefore, the effects of individual B. subtilis volatiles on the changes in motility and antibiotic resistance were tested. We selected seven commercially available VOCs of the ~30 VOCs [44] , and examined VOC-mediated induction of swarming motility and the antibiotic resistance phenotype. The screenings showed that exposure to 2,3-BD, one of the primary ketones synthesized in B. subtilis GB03, and GA, the second-most synthesized acid from B. subtilis GB03 [44] , reproducibly reduced swarming motility ( Fig. 4a ). These VOCs elicited a resistance response to ampicillin that was similar to the total VOC-induced phenotype in both strains ( Fig. 4b ). The level of antibiotic resistance induced by 3M1BOH and 2M1PAOL was dramatically different in the two strains ( Fig. 4b ). Variations in the architecture of strains can influence motility and biofilms [30] , and it is possible that the architecture of these E. coli strains contributes to their different responses to VOCs. These data strongly suggest that VOCs, in particular 2,3-BD and GA, modulate swarming motility and antibiotic resistance in E. coli cells. 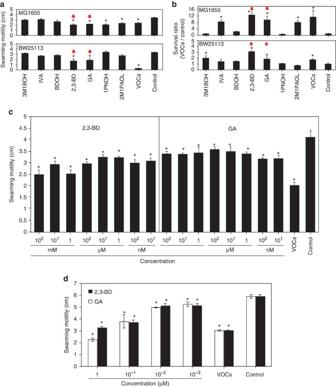Figure 4: Identification and characterization of individual VOCs affectingE. coliphenotypes. Effect of individual VOCs on (a) swarming motility and (b) ampicillin resistance inE. coliMG1655 and BW25113 (n=3,P=0.05). The antibiotic resistance phenotype was expressed as the survival ratio of VOC-treated and VOC-untreatedE. coligrown on ampicillin. Control represents no VOC treatment. Determination of effective concentration of individual VOCs by (c) natural vaporization (gaseous phase) or by (d) direct addition (aqueous phase). Asterisks (*) indicate statistically significant data (P=0.05) and arrowheads indicate individual VOCs that show the same phenotype as total VOCs in both BW25113 and MG1655 cells. Error bars are defined as s.e.m. Figure 4: Identification and characterization of individual VOCs affecting E. coli phenotypes. Effect of individual VOCs on ( a ) swarming motility and ( b ) ampicillin resistance in E. coli MG1655 and BW25113 ( n =3, P =0.05). The antibiotic resistance phenotype was expressed as the survival ratio of VOC-treated and VOC-untreated E. coli grown on ampicillin. Control represents no VOC treatment. Determination of effective concentration of individual VOCs by ( c ) natural vaporization (gaseous phase) or by ( d ) direct addition (aqueous phase). Asterisks (*) indicate statistically significant data ( P =0.05) and arrowheads indicate individual VOCs that show the same phenotype as total VOCs in both BW25113 and MG1655 cells. Error bars are defined as s.e.m. Full size image Determination of effective VOC concentrations for phenotypes Our data clearly showed an effect of total and individual airborne VOCs from physically separated bacteria on the phenotypes of receiver bacteria. However, how VOCs, which are gaseous molecules, affect the receiver bacteria is not clear. It is possible that gaseous VOCs are solubilized in the culture media of E. coli , and the amount affects their function. Therefore, a determination of the working concentrations of 2,3-BD and GA that are effective for the bacterial phenotypes will indicate the relevance of two airborne VOCs on the physiology of physically separated bacteria. To determine the index of the VOC effect, we measured the effective concentration of 2,3-BD and GA by natural vaporization of B. subtilis VOCs to E. coli cells. For this purpose, swarming motility was measured after treatment with different concentrations (10 nM to 100 mM) of 2,3-BD or GA for 16 h. As seen in Fig. 4c , application of 10 nM of 2,3-BD or GA by the method described in Fig. 1 modified the swarming motility (~22−25% decrease compared with non-treated controls), whereas total VOCs decreased motility by ~50%. This information defines tentative volatility as the percentage change of motility by time of VOC treatment (% h −1 ). Therefore, the volatility of 2,3-BD and GA is ~22–25% h −1 , and ~50% h −1 for total VOCs. To determine the amount of 2,3-BD or GA in the media that directly affects the phenotype, either 2,3-BD or GA from 1 nM to 1 μM was directly added to the E. coli cell cultures. With 1 nM of 2,3-BD or GA, there was a linear decrease in swarming motility. At 1 μM of 2,3-BD or GA, there was a volatility of ~62% h −1 or ~45% h −1 , respectively ( Fig. 4d ). In those conditions, the growth of E. coli was not affected by the increased concentration of individual VOCs ( Supplementary Fig. S3 ). E. coli were resistant to ampicillin, even when picomolar final concentrations of 2,3-BD and GA were added ( Supplementary Fig. S4 ). These results indicate that both gas and liquid phases of VOCs affect motility and susceptibility to antibiotics when receiver bacteria are treated with VOCs in concentration ranges of pM to μM, which are physiologically relevant concentrations. Mechanistic studies on the VOC-induced pathways The data indicated that VOCs affect the expression of groups of genes related to cellular phenotypes of bacteria. Another question is how VOCs affect the phenotypes. Because the cellular pathways are generally mediated by complex systems, it might be postulated that a master regulatory gene controls the VOC-mediated phenotypes by modulating transcription factors. To identify the master regulators, knockout mutants of VOC-modulated genes that no longer exhibited VOC-related phenotypes, such as swarming motility or antibiotic resistance, were selected for further investigation. VOCs exerted no change in the swarming motility of five candidate knockout mutants ( ybgL , ybjL , ypdB , ykg and yfbK ; Fig. 2e , Table 1 ). When the effect of VOCs on the antibiotic resistance of these mutants was studied, only the absence of ypdB resulted in reduced antibiotic resistance ( Fig. 5a ). The ypdB mutation showed the same effect on bacterial growth as in wild-type cells ( Fig. 5b ). 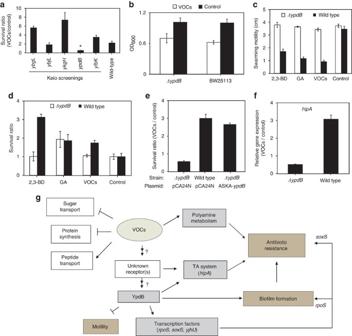Figure 5: Master regulation of VOC-mediated phenotypes by theypdBgene product. (a) Identification of VOC-regulated genes involved in antibiotic resistance. Survival ratio of VOC-treated to VOC-untreated Keio collection mutants grown in the presence of ampicillin (n=3). Asterisk (*) indicates the statistical significance (P=0.05). (b) Growth phenotypes of wild-type andypdBknockout by VOCs. The growth (OD600) was monitored by the absence or presence of VOCs by natural vaporization. Comparison of the effect of 2,3-BD and GA on swarming motility (c) and antibiotic resistance (d) in aypdB-knockout and wild-typeE. coli. (e) Survival ratio of VOC-treated to VOC-untreated cells in aypdBknockout, the complemented knockout and wild-type cells grown in the presence of ampicillin. (f) Relative change inhipAexpression with and without VOC treatment in wild-typeE. coliandypdB-knockout cells (n=3,P=0.05). (g) Model for VOC-mediated changes toE. coliphysiology. The model is based on data from this study and previous reports. Error bars are defined as s.e.m. Figure 5: Master regulation of VOC-mediated phenotypes by the ypdB gene product. ( a ) Identification of VOC-regulated genes involved in antibiotic resistance. Survival ratio of VOC-treated to VOC-untreated Keio collection mutants grown in the presence of ampicillin ( n =3). Asterisk (*) indicates the statistical significance ( P =0.05). ( b ) Growth phenotypes of wild-type and ypdB knockout by VOCs. The growth (OD 600 ) was monitored by the absence or presence of VOCs by natural vaporization. Comparison of the effect of 2,3-BD and GA on swarming motility ( c ) and antibiotic resistance ( d ) in a ypdB -knockout and wild-type E. coli . ( e ) Survival ratio of VOC-treated to VOC-untreated cells in a ypdB knockout, the complemented knockout and wild-type cells grown in the presence of ampicillin. ( f ) Relative change in hipA expression with and without VOC treatment in wild-type E. coli and ypdB -knockout cells ( n =3, P =0.05). ( g ) Model for VOC-mediated changes to E. coli physiology. The model is based on data from this study and previous reports. Error bars are defined as s.e.m. Full size image Swarming motility in the ypdB knockout was similar to the untreated control, and did not show any significant change following exposure to 2,3-BD, GA or total VOCs ( Fig. 5c ). The survival ratio of the ypdB -knockout cells was similar to that in wild-type cells in the absence of VOCs. However, the survival ratio of ypdB -knockout cells was lower than that in wild-type cells exposed to 2,3-BD and total VOCs ( Fig. 5d ). VOC-induced antibiotic resistance was eliminated by the ypdB deletion and complemented by ectopic induction of ypdB in the knockout strain ( Fig. 5e ). The expression of hipA was severely reduced in the ypdB knockout ( Fig. 5f ), which suggests that the ypdB gene product might function as an upstream activator or transcription factor for hipA expression. Therefore, ypdB may be the master regulator of VOC-mediated effects in E. coli . There have been many reports that chemicals work as signals for the transcription of specific genes [45] . We hypothesized that gene-expression changes induced by VOCs reflect the modified activity of transcription. To test our hypothesis, we examined the transcription activity (that is, promoter activity) of some genes that are upregulated by VOCs. For this purpose, chromosomal promoter-green fluorescent protein (GFP) fusions of three genes ( ycfR , aaeX and hyaF ) that show >3-fold changes in transcript levels induced by VOCs ( Fig. 1 ) were generated. Then, the expression of hybrid-GFP proteins in E. coli cells exposed to B. subtilis VOCs and untreated controls (no B. subtilis ) were measured. All selected genes showed increased expression of GFP in response to B. subtilis VOCs ( Supplementary Fig. S5 ), suggesting that VOCs could affect the transcription of target genes by modulating promoter activity. We searched for transcription-related factors that were related to the phenotypes. For this purpose, we introduced a fluorescent promoter library [46] for the screening of factors on the phenotypes. From the library, 60 available promoter reporters were selected as transcription-related libraries after filtering by keywords of transcription or DNA-binding transcription regulation using both EcoCyc [47] and gene descriptions of microarray data ( Supplementary Table S4 ). A 96-well plate was used to screen reporters with natural vapourization from 1 μM of 2,3-BD or GA or B. subtilis VOCs (from 10 [5] cells) for 14 h at 37 °C. The promoter activity as fluorescence from E. coli promoter reporters was monitored as fluorescence/OD 600 . From the results of 60 different promoters ( Supplementary Table S4 ), the activity of three different genes ( yjhU , soxS or rpoS ) was reproducibly induced by all tested VOCs (2,3-BD, GA and B. subtilis VOCs) ( Table 2 ). Therefore, these genes could be either upstream or downstream genes of VOC-mediated responses by the ypdB product. This hypothesis was further validated by analysis of the steady-state level of those transcription factors using RT–qPCR in the presence or absence of ypdB or individual VOCs (2,3-BD). We found that the levels of three genes ( soxS , yjhU and rpoS ) were increased by treatment with 2,3-BD ( Table 2 ). The gene expression of all targets decreased in the absence of ypdB , suggesting that those genes are activated by the ypdB gene product and are located downstream of ypdB . These data indicate that the ypdB product and its downstream transcription factors mediate the regulatory cascades of VOC-induced phenotypes. Table 2 Effect of VOCs on promoter activity * or transcript level † . Full size table Our study showed that airborne VOCs are important molecules in sensing distant bacteria even without physical contact. We found that gaseous VOCs released from B. subtilis severely affect neighbouring Gram-negative bacteria either as gas or liquid molecules, resulting in a change of gene-expression profiles that alter both motility and antibiotic-resistance phenotypes. The VOC-mediated motility phenotype is conserved in both Gram-negative ( B. glumae and P. aeruginosa ) and Gram-positive ( P. polymyxa ) bacteria. The 2,3-BD and GA from total VOCs of emitter bacteria are major signalling molecules that affect motility, antibiotic resistance [48] and increased biofilm formation (a general trait relating to antibiotic resistance [49] and rpoS mediation [50] ) ( Supplementary Fig. S6 ). The VOC-mediated phenotypes are linked to a previously uncharacterized ypdB gene product and downstream transcription factors. Therefore, these VOC signalling cascades of ypdB /transcription factors could rapidly alter gene-expression profiles and result in multiple phenotypic changes involved in bacterial growth and adaptation to environmental stresses. VOCs from emitting bacteria might function as effector molecules that target transcription-related factors of interacting bacteria, resulting in the rapid alteration of gene-expression profiles. This seemed to be an energetically efficient way to simultaneously control many genes. This hypothesis was supported by the results that VOCs increased the promoter activity of genes that were upregulated in the microarray analysis ( Fig. 5a ), including several known stress-responsive transcription factors ( soxS , rpoS and yhjU ). The gene expression of such transcription factors could function as the downstream genes to ypdB , considering the decreased gene expression in the absence of ypdB when 2,3-BD is present ( Fig. 5 ). Our results indicate that VOC-mediated phenotypes are mediated by the master regulation of the ypdB gene product and its downstream transcription factors. Therefore, the genes identified in this study could be useful as targets for the development of antimicrobials. Although many bacteria produce VOCs [25] , little is known about their physiological functions. Several recent reports indicate that bacteria are responsive to VOCs, including ammonia. Ammonia is a valuable nutrient for the production of proteins and nucleic acids for bacteria. The Burgess group recently showed that the soil bacterium Bacillus licheniformis was sensitive to the presence of ammonium sulphate [51] , which is metabolized and converted to ammonia, resulting in the induction of biofilm formation. The mechanisms underlying the roles played by VOCs in bacterial communication were unknown. Ghigo and colleagues [14] also showed that ammonia from E. coli influenced antibiotic resistance in aerially exposed Gram-positive and Gram-negative bacteria. The authors discovered a previously uncharacterized antibiotic-resistance mechanism and showed that this effect contributed to the induction of ammonia- and polyamine-related genes during the stationary phase. In our unpublished preliminary results, we did not identify ammonia as a major signal from B. subtilis as a source of VOCs. Therefore, we did not perform experiments with polyamine as a major VOC. This suggests that the source of the two VOCs was completely independent from volatile amines. Our study provides the first evidence of a mechanism underlying VOC-modified gene expression in interacting bacteria each other. The volatility of gaseous materials is an important factor for understanding the fate of individual VOCs. We determined the tentative volatility of 2,3-BD and GA as the percentage change of motility by time of VOC treatment (% h −1 ) ( Fig. 4 ), which was ~62% or 45% h −1 for 2,3-BD or GA, respectively. However, this is not a general index and many people use Henry’s constant (k° H , mol kg −1 ·bar) instead, which states the amount of gas that dissolves in liquid at equilibrium and constant temperature. By comparing the k° H in water at 25 °C, the volatility of 2,3-BD (k° H =74) [52] is much higher than that of GA (k° H =9,000) [53] . These data suggest that 2,3-BD will most likely evaporate, whereas GA is effectively dissolved in water. In our study, the solubilizing amount of individual VOCs was not a decisive factor for phenotypes, considering that both gas and liquid phases of VOCs at pM to μM concentrations were sufficient for the phenotypes. Using gas chromatography-mass spectrometry solid phase microextraction (GC-MS SPME) profiling of rhizobacterial volatiles, 2,3-BD was released at 77 μg per 24 h, whereas GA was released at ~1 μg from B. subtilis GB03 (ref. 44 ). The release of 2,3-BD was less in Gram-negative bacteria, such as E. coli (DH5α) (14 μg per 24 h) and Pseudomonas fluorescens 89B61 (7 μg per 24 h), whereas Bacillus amyloliqefaciens IN937a released 38 μg per 24 h. The production of the large amount of 2,3-BD from Bacillus species was still an enigma, but we showed that 2,3-BD (even with lower amounts as either gas or liquid phase) affects specific biological processes. The VOC 2,3-BD occurs naturally in alcoholic beverages and is added to some foods to give a buttery flavour and aroma. Food flavourings containing 2,3-BD are used in microwave popcorn and other snack foods, pet foods, candies, baked goods and other food products [54] . It is an antimicrobial compound produced by bacteria such as lactic acid bacteria, which produce antimicrobial compounds including hydrogen peroxide, carbon dioxide, 2,3-BD, various uncharacterized compounds and high molecular mass compounds, such as bacteriocin [55] . However, its effectiveness as an antimicrobial agent among bacteria seems not to be a generalized phenomenon, but is context dependent. For example, 5.8–29 mM of 2,3-BD in skimmed milk is more effective against Gram-negative bacteria than Gram-positive bacteria, with lactobacilli having the highest resistance [55] , [56] . The minimum-inhibitory concentration of 2,3-BD among bacteria differs according to pH (ref. 55 ). In our study, E. coli growth was severely decreased by the addition of 2,3-BD (>1 mM) ( Supplementary Fig. S3 ). This appeared to be the minimum susceptible concentration of 2,3-BD as antibiotics for E. coli , which are matched to the Hedgecock and Jay’s results [55] , [56] . However, at extremely low dosage (nM to μM concentration) of 2,3-BD, the effect is completely reversed to that of higher dosage. The low amount of 2,3-BD that is effective to induce VOC-mediated phenotypes is comparable to the concentration of 2,3-BD in wines for the taste threshold: 0.2 mg l −1 (2.4 μM) for Chardonnay wine, 0.9 mg l −1 (10.8 μM) for Pinot Noir and 2.8 mg l −1 (33.6 μM) for Cabernet Sauvignon [57] . How a low dosage of 2,3-BD affects bacterial diversity is related to human health, although a higher dose of 2,3-BD induces respiratory toxicity in mammals [58] , [59] , [60] . One of the easy samples will be the wine microbiome [61] . We could identify the negative or positive selection pressure of bacterial diversity using 2,3-BD. GA is produced as an intermediate of the glyoxylate cycle, which is a variation of the tricarboxylic acid cycle that synthesizes carbohydrates from C2 compounds, such as ethanol and acetate [62] . This product as a VOC occurs in many bacteria [44] , [62] , [63] such as Bacillus , E. coli and Rhodobacter species. Therefore, our results that GA functions as a signal molecule to modulate multiple phenotypes might be correlated with general bacterial acetate metabolism. Further work will identify VOC-responsive targets in the pathway, and these will be good candidates for controlling the antibiotic-resistance pathways. Although 2,3-BD and GA were effective at modulating the expression profiles of genes related to bacterial motility and antibiotic resistance in E. coli , many biological questions remain unanswered. These include the identification of additional biogenic volatile molecules and the complete mechanistic behaviour of long-range interactions. Similar to the recent progress made in identifying the interactions mediated by indole [6] , which was a known bacterial product for over 100 years, the biological roles of VOCs are only now beginning to be elucidated. However, it is clear that the VOC-mediated pathways are an important method of communication between physically separated bacteria. They induce changes in gene expression that may facilitate survival, such as increased antibiotic resistance. Therefore, VOC-mediated bacterial communication may promote modulation of self-defence phenotypes and motility changes in physically separated bacteria. Strains B. subtilis 168 ( [24] ) (Bacillus Genetic Stock Center), E. coli MG1655 ( [31] ) or BW25113 ( [29] ) were used as parental strains. For the mutant analysis, Keio collections [28] were used. B. glumae BGR1 (ref. 61 ), P. aeruginosa PA14 (ref. 64 ) or P. polymyxa E681 (ref. 65 ) were used for the swarming motility assay. Chemicals High-purity individual VOCs (>99%) were purchased from Sigma-Aldrich. Each VOC was expressed as an acronym: 3M1BOH (3-methyl-1-butanol), IVA (3-methylbutanoic acid; isovaleric acid), BDOH (butane-2,3-diol), 2,3-BD (butane-2,3-dione; 2,3-butanedione or diacetyl), GA (oxoethanoic acid or glyoxylic acid), 1PNOH (pentan-1-ol; 1-pentanol) and 2M1PAOL (2-methyl-1-propanol). Cell culture and exposure to VOCs To perform the experiments on the effect of B. subtilis , VOCs on E. coli , B. glumae , P. aeruginosa or P. polymyxa cells on the I-plate (Falcon, No. 351003) assay were used. Each culture was prepared by inoculating B. subtilis or E. coli MG1655, BW25113, B. glumae , P. aeruginosa or P. polymyxa in different media as follows: for B. subtilis and P. polymyxa , TSB (Difco); for E. coli and B. glumae , LB broth; for P. aeruginosa , Nutrient Broth (NB). The culture condition for each bacteria was different: E. coli , B. subtilis and P. aeruginosa were cultured at 37 °C for 16−24 h; B. glumae and P. polymyxa were cultured at 30 °C for 24−48 h. For further analysis of VOC effects, ~10 [5] cells of each bacteria were spread onto TSB-, LB- or NB-agar plates. All growth was monitored by using Ultrospec 2100 pro (AP Biotech). Transcriptome analysis The analysis was performed using E. coli chips described in the KRIBB Genome Encyclopedia of Microbes [66] , except that genes showing VOC-dependent differences in expression levels of ≥2-fold or ≤0.5-fold were considered to be differentially expressed genes. Clustering analysis was performed by MultiExperiment Viewer [67] . Construction of single-copy promoter-GFP fusions The preparation of backbone plasmid pGEM-T-GFPCm was performed in three consecutive steps. First, the GFP region was amplified from pDSK-GFPuv [68] using primers GFP-F. Second, the chloramphenicol (Cm) cassette fragment was amplified using primers GFP-P1-F and GFP-P2. Finally, GFP-Cm products were prepared by the fusion PCR method as described in a previous report [69] , followed by cloning of the PCR product into the pGEM-T-easy vector (Promega). This resulted in pGEM-T-GFPCm. Chromosomal ycfR , aaeX or hyaF promoter fusions were performed by E. coli single-gene knock-out method [29] , with pGEM-T-GFPCm and the following primers for each gene: ycfR -HL, ycfR -HR, aaeX -HL, aaeX -HR, hyaF -HL and hyaF -HR. The construction was confirmed by the gene-specific primers ycfR -192-F, aaeX -76-F and hyaF -181-F, or the universal primer GFP-R. Identification of transcription factors modulating VOC phenotypes The screening of transcription-related factors affected by VOCs was performed using a library of fluorescent transcriptional reporters of E. coli (Open Biosystems) [46] . By using the term ‘transcription factor or DNA-binding transcription regulator’ in both EcoCyc and microarray data, 60 available reporter genes were selected ( Supplementary Table S4 ). Overnight cultures of E. coli cells containing individual transcriptional reporters were inoculated into fresh LB media (1/100 dilution) containing kanamycin (50 μg ml −1 ) on 96-well plates in the condition of vaporization of 2,3-BD or GA (1 μM final) for 14 h at 37 °C. The promoter activity was monitored and analyzed [68] with 2104 EnVision multilabel plate readers (PerkinElmer). The normalized promoter activity (fluorescence/OD 600 ) to control vector of the reporter system was analysed for all 64 genes from triplicate experiments ( n =3, P =0.05). Swimming and swarming motility assay For swimming motility assays, TSB- or LB-agar (0.3%) plates were separately prepared in either side of I-plate. B. subtilis or E. coli (~10 5 cells) were spread onto either TSB- or LB-agar plate, respectively, followed by incubation at 37 °C for 12 h and photography of results. The swarming motility assay was performed using a different recipe for the growth of receiver bacteria on the plate: LB agar (LB broth+0.5% agar+0.5% glucose) for E. coli and B. glumae ; NB agar (NB broth+0.5% agar+0.5% glucose) for P. aeruginosa ; TSB agar (TSB+0.9% agar) for B. subtilis and P. polymyxa . For the assay, B. subtilis (~10 5 ), cells were spread onto TSB agar, and bacteria were inoculated onto species-specific agar described above. The plates were incubated at either 30 or 37 °C for 12–48 h and photographed. To observe the effect of individual gas-phase VOCs, the specified concentration (indicated in each Figure legend) of 2,3-BD or GA solution was dropped onto the TSB-agar plate instead of emitter B. subtilis cells. Screening of bacterial antibiotic resistance by VOC treatment To identify bacterial antibiotic-resistant phenotypes in response to VOC treatment, E. coli cells were subjected to PM analysis (PM plates No. 11–20). E. coli MG1655 cells were treated with or without total VOCs from B. subtilis (~10 5 cells) for 16 h at 37 °C. The resulting cells were scraped, diluted to OD 600 =0.3 in PM media and subjected to analysis by PM for 24 h at 37 °C (ref. 39 ). Antibiotic-resistance assays To validate VOC-mediated resistance to both ampicillin and tetracycline, E. coli cells with or without vaporization of B. subtilis VOCs were cultured on I-plate for 12 h. The cells were collected by scraping and diluted to OD 600 =0.1 in LB broth. Either ampicillin (100 μg ml −1 ) or tetracycline (10 μg ml −1 ) was added to the culture and then grown further for 3 h at 37 °C with vigorous shaking. A fraction of the cultures was spread on LB plates, and the survival ratio was determined by counting the colonies on LB plate. The survival ratio of VOCs-treated and non-VOCs-treated were compared from triplicate experiments ( n =3, P =0.05). Reverse transcription quantitative PCR Total RNA from E. coli was prepared using RNeasy plus mini kit (Qiagen) according to the manufacturer’s protocol. cDNA synthesis was performed as follows: total RNA (0.5 μg) was used for the template for the RT reaction using ReverTraAce qPCR RT Master Mix with gDNA Remover (Toyobo) according to a previous report [68] . A CFX connector real-time qPCR system (Bio-Rad) was used for RT–qPCR. Reaction mixtures consisted of cDNA, iQ SYBR Green Supermix (Bio-Rad) and 1 pM of each primer set listed in Supplementary Table S6 . The PCR parameters were as follows: initial polymerase activation, 3 min at 95 °C, 40 cycles of 10 s at 95 °C, 10 s at 60 °C and 30 s at 72 °C. Conditions were determined by comparing threshold values in a series of dilutions of the RT product, followed by a non-RT template control and a non-template control for each primer pair. Relative RNA levels were calibrated and normalized to the level of rrsB (16S rDNA) RNA. Statistical analysis The statistical analyses were performed as previously described [19] using JMP software. Error bars are defined as s.e.m. in all data analysis. How to cite this article: Kim, K.-S. et al . Interspecific bacterial sensing through airborne signals modulates locomotion and drug resistance. Nat. Commun. 4:1809 doi: 10.1038/ncomms2789 (2013).